High-efficiency ballistic electrostatic generator using microdroplets The strong demand for renewable energy promotes research on novel methods and technologies for energy conversion. Microfluidic systems for energy conversion by streaming current are less known to the public, and the relatively low efficiencies previously obtained seemed to limit the further applications of such systems. Here we report a microdroplet-based electrostatic generator operating by an acceleration-deceleration cycle (‘ballistic’ conversion), and show that this principle enables both high efficiency and compact simple design. Water is accelerated by pumping it through a micropore to form a microjet breaking up into fast-moving charged droplets. Droplet kinetic energy is converted to electrical energy when the charged droplets decelerate in the electrical field that forms between membrane and target. We demonstrate conversion efficiencies of up to 48%, a power density of 160 kW m −2 and both high- (20 kV) and low- (500 V) voltage operation. Besides offering striking new insights, the device potentially opens up new perspectives for low-cost and robust renewable energy conversion. Electrostatic generators historically precede electromagnetic generators, and are still used for high voltage applications [1] . Their working principle is invariably based on the transport of a solid or liquid medium with adsorbed charge to a location of higher electrical potential by continuous application of a mechanical force, typically with low efficiency [2] . Microfluidics technology stands out by its versatility and wide applicability, especially when using electrical control methods [3] , [4] , [5] , [6] , [7] , [8] , [9] , [10] . Micro- and nanofluidic energy conversion systems have recently been studied using the streaming potential phenomenon. Maximal conversion efficiencies of 3–5% were obtained in nanofluidic channels [11] , [12] and nearly 11% in a microjet system [13] , [14] . Here, we demonstrate a novel principle for fluidic energy conversion, which we call ballistic energy conversion. The system can be classified as an electrostatic generator (like the van de Graaff generator), but unlike all other electrostatic generators is based on an acceleration/deceleration cycle, effected by jetting high-velocity charged droplets to a target at high potential. Following this principle, we demonstrate that the strong reduction of friction enables conversion efficiencies of almost 50% and a power density of maximally 160 kW m −2 while at the same time allowing for an extremely simple design. Device and working principle The generator is shown in Fig. 1a,b . A high-speed (>10 m s −1 ) water microjet is formed by forcing water (by ~100 kPa overpressure) through a micropore etched in an ultrathin silicon nitride membrane ( Supplementary Figs 1 and 2 ). The jet breaks up into a stream of droplets by the Rayleigh–Plateau instability ( Fig. 1c ) [15] , [16] , [17] . The droplets carry a net positive ionic charge. This charge originates from advection of the positive mobile ions in the electrical double layer (EDL) of the membrane, (the streaming current phenomenon) but as we demonstrate can be strongly increased by induction, by applying a negative potential to the metal ‘guard ring’ located close to the pore exit. The droplets travel through the air towards a metal target that acquires a high electrical potential by charge accumulation owing to droplet impact. Along the droplet trajectory, the high electrical field between target and jet decelerates the droplets at ~10 4 g. As the droplets move to a location of higher electrical potential, their kinetic energy is directly converted into electrical energy (‘ballistic energy conversion’) due to the force balance ma = −qE with m and q droplet mass and charge, a acceleration and E electrical field (for the moment neglecting air friction). Current is drawn from the high potential target to do useful work. The function of the guard ring is to modify the local electrical field: when it is grounded, it prevents induction of negative charge in the jet by the positively charged target, and when it is held at negative potential, it induces additional positive ionic charge in the jet. It should be emphasized that the induction process by the guard ring does not consume energy, as no current flows through the guard ring under normal operation. Typical experimental parameters are listed in Supplementary Table 2 . 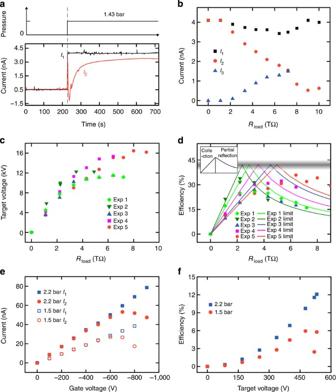Figure 2: Experimental results using 10 μm diameter pores. (a) Upstream and downstream current on application of pressure. The guard ring was grounded during this experiment. (b) Upstream, downstream and guard ring current with increasing value of the load resistance. (c) Generated target voltage as function of load resistance for different upstream currents. (d) Conversion efficiency as a function of load resistance for different values of the upstream current. Experimental values (symbols) and theoretical predictions (lines) are shown, as well as the theoretical maximum efficiency of 37–43% (depending on flow rate). (e,f). High current, low-voltage operation. (e) Current as function of gate voltage. (f) Efficiency of the experiments shown undereas a function of generated target voltage. For data seeSupplementary Table 3. The system operates by physics that fundamentally differs from the physics governing both classical fluidic electrokinetic energy conversion systems and electrostatic generators [3] , [4] , [18] , [19] , [20] . It was inspired by prior work on microjet energy conversion [13] , [14] , [21] . However, the electrostatic induction of charge allows operation independently of the EDL on the membrane surface, enabling an increased droplet charge density and thus a lower target voltage. This offers great advantages for future applications, as will be discussed below. We first report on experiments using 10 μm diameter pores, where we obtain a maximal efficiency of 36% and show operation both in high voltage, low-current mode and low voltage, high-current mode. 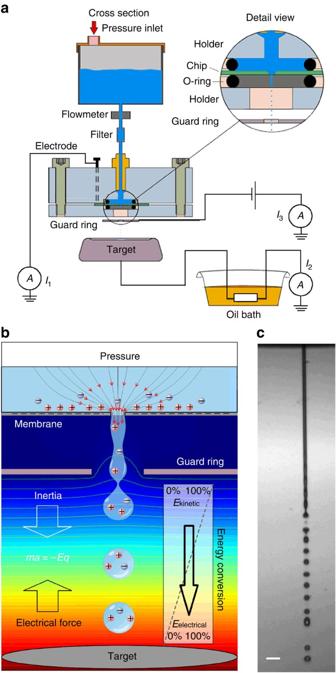We then show measurements on an optimized (from the physical model) system with a 30-μm diameter pore, where we obtain a maximal efficiency of 48%. Figure 1: Concept of energy conversion and set-up. (a). Experimental set-up. Aqueous solution is forced by applied air pressure through a 10 or 30 μm diameter circular pore in a 500-nm-thick silicon nitride membrane. A platinum electrode sputtered on the backside of the chip (30 μm pore experiments) or an inserted platinum wire (10 μm pore experiments) was connected to a picoammeter (Keithley 6485). A microjet is formed that breaks up in a droplet stream. The droplets travel through the air and arrive on a metal target placed at 7.5–25 mm distance from the pore opening. The target is connected to electrical ground via a high-load resistance (typically 1–10 TΩ,Supplementary Table 1). A metal guard ring with an opening of 2 mm diameter is placed at 1.5 mm (10 μm pore) or 5.0 mm (30 μm pore) from the pore exit and maintained at ground potential, or at a negative potential for inductive droplet charging. The current can be measured between ground and the platinum reservoir electrode (denotedI1), between target and ground (I2) and between metal guard ring and ground (I3). (b). Conceptual illustration of the conversion principle. Water is accelerated to form a microjet that breaks up into charged droplets. On their air trajectory towards the target, the droplets are decelerated by the electrical force, converting kinetic energy into electrical energy. The background colour from red to blue indicates the voltage distribution from high to low, the lines denote equipotentials. (c) Photomicrograph of the microjet from the 10 μm pore taken by double iLIF illumination (Supplementary Figs 10 and 11). Scale bar, 40 μm. Figure 1: Concept of energy conversion and set-up. ( a ). Experimental set-up. Aqueous solution is forced by applied air pressure through a 10 or 30 μm diameter circular pore in a 500-nm-thick silicon nitride membrane. A platinum electrode sputtered on the backside of the chip (30 μm pore experiments) or an inserted platinum wire (10 μm pore experiments) was connected to a picoammeter (Keithley 6485). A microjet is formed that breaks up in a droplet stream. The droplets travel through the air and arrive on a metal target placed at 7.5–25 mm distance from the pore opening. The target is connected to electrical ground via a high-load resistance (typically 1–10 TΩ, Supplementary Table 1 ). A metal guard ring with an opening of 2 mm diameter is placed at 1.5 mm (10 μm pore) or 5.0 mm (30 μm pore) from the pore exit and maintained at ground potential, or at a negative potential for inductive droplet charging. The current can be measured between ground and the platinum reservoir electrode (denoted I 1 ), between target and ground ( I 2 ) and between metal guard ring and ground ( I 3 ). ( b ). Conceptual illustration of the conversion principle. Water is accelerated to form a microjet that breaks up into charged droplets. On their air trajectory towards the target, the droplets are decelerated by the electrical force, converting kinetic energy into electrical energy. The background colour from red to blue indicates the voltage distribution from high to low, the lines denote equipotentials. ( c ) Photomicrograph of the microjet from the 10 μm pore taken by double iLIF illumination ( Supplementary Figs 10 and 11 ). Scale bar, 40 μm. Full size image Energy conversion efficiencies For a typical experiment with a 10-μm diameter pore and demineralized water, Fig. 2a shows the upstream current I 1 , from grounded reservoir electrode to jet, and the downstream current I 2 , from target to ground. When jetting starts at t =220 s, charge directly flows out of the reservoir as indicated by I 1 . The exponential increase of I 2 is determined by the electrical RC time (product of target capacitance C and load resistance R). The steady-state difference between both currents is caused by the reflection of charged droplets from the target at high potential ( Supplementary Fig. 3 ), landing on the grounded guard ring and generating current I 3 . Figure 2b displays the currents I 1 , I 2 and I 3 for a typical measurement in which the load resistance is increased in steps of 1 TΩ. I 1 remains approximately constant, while I 2 decreases with load resistance and I 3 increases from initially zero. Figure 2c plots the target voltage, calculated as the product of harvested current I 2 and load resistance as V target =I 2 ·R load against load resistance for a number of experiments. The target voltage increases with load resistance up to between 10 and 16 kV, where it is found to saturate. The conversion efficiency from mechanical to electrical energy, Eff=I 2 ·V target /(p·Q) , with p (Pa) the applied reservoir pressure and Q (m 3 s −1 ) the volumetric flow rate. The conversion efficiency was found to increase with load resistance ( Fig. 2d ), for 10 μm pores reaching a typical efficiency around 33% with a highest value of 36%. Figure 2: Experimental results using 10 μm diameter pores. ( a ) Upstream and downstream current on application of pressure. The guard ring was grounded during this experiment. ( b ) Upstream, downstream and guard ring current with increasing value of the load resistance. ( c ) Generated target voltage as function of load resistance for different upstream currents. ( d ) Conversion efficiency as a function of load resistance for different values of the upstream current. Experimental values (symbols) and theoretical predictions (lines) are shown, as well as the theoretical maximum efficiency of 37–43% (depending on flow rate). ( e , f ). High current, low-voltage operation. ( e ) Current as function of gate voltage. ( f ) Efficiency of the experiments shown under e as a function of generated target voltage. 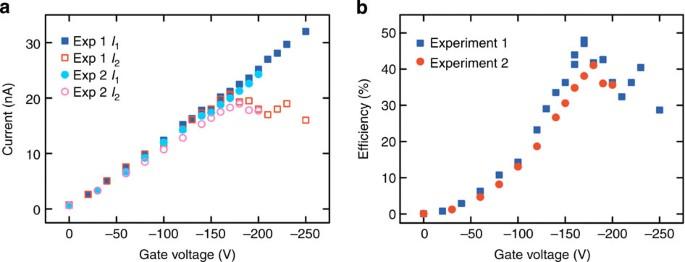Figure 3: Two experiments using a 30-μm diameter pore. (a). CurrentsI1andI2as a function of gate voltage. (b) Efficiency as a function of gate voltage with a 1.01-TΩ load resistance. Applied pressure 1.38 bar, average flow rate 6.55 μl s−1, solution 10 mM KCl, target distance 2.5 cm (experiment 1) and 2.0 cm (experiment 2). For data see Supplementary Table 3 . Full size image An analysis of the conversion mechanism indicates two distinct phases. In the first phase, water is accelerated and droplets are formed during conversion of input power p·Q into droplet kinetic power ½ Q·ρv 2 (with ρ the density of water and v the droplet velocity). Here power is lost by viscous friction near the pore and by the interfacial energy needed to form the jet. From the measured droplet velocity at jet break-up, we found that these combined losses amount to ~52% for 10 μm pores ( Supplementary Figs 4 and 5 ). In the second phase, droplets are decelerated along their trajectory by the force exerted by the electrical field E on the droplet charge q with the force balance ma=−qE−F fr where F fr is the air friction force. We estimate the frictional power loss along the air trajectory as 17% ( Supplementary Note 1 ). For 10 μm pores, a maximum efficiency of 40% is therefore predicted for the entire conversion (0.83 × 0.48), in good agreement with our experimentally observed maximum efficiency of 36%. The trajectory droplet velocity decrease was experimentally documented ( Supplementary Note 1 ). A more detailed paper on the theoretical optimization of the system is in preparation. On the basis of the acceleration/deceleration mechanism, we expect two regimes of operation, which can be observed in Fig. 2c,d . At low values of the load resistance, target potential V target = I 2 ·R load = I 1 ·R load is low and the kinetic energy of the droplets is only partially converted into electrical energy. In this ‘collection regime’, the target potential linearly increases with the load resistance as does the efficiency Eff =(I 1 ) 2 ·R load /(pQ). Increasing the load resistance, the target potential at constant I 2 = I 1 will reach a value where droplets will only just be able to reach the target with the kinetic energy available. The highest potential that can be reached with 10 μm pores at 40% efficiency is V opt =0.40 ·pQ/I 1 is generated at load resistance R opt =V opt /I 1 . In various experiments V opt varied between 11.5 and 17 kV ( Fig. 2c ). When the resistance is further increased, an increasing fraction of the droplets is observed to be reflected from the target ( Supplementary Fig. 3 ). In this ‘partial reflection regime’ I 2 becomes progressively smaller than I 1 with increasing R load ( Fig. 2b ). Assuming that all droplets have identical charge to mass ratio, I 2 in this regime will be inversely proportional to R load since V target =V opt =I 2 ·R load and the efficiency equals 0.40· R opt /R load . The expected efficiency curves as plotted in Fig. 2d are in good agreement with the observations. We attribute the observed gradual transition between both operating regimes to a spread in the droplet charge over mass ratio q/m . Typically, about 20% of the droplet charge is lost at maximal efficiency ( Supplementary Fig. 6 ), causing it to be slightly lower than the theoretical expected value of 40%. A variation in the droplet size at jet break-up was indeed observed ( Supplementary Fig. 7 ). Some of the efficiency values observed in the partial reflection regime exceed the theoretical predictions, which can be explained by variations in the upstream current I 1 (see for example, Fig. 1b ). A distance of 10–15 mm between membrane and target was found to be optimal ( Supplementary Fig. 8 ), since it minimized air friction loss while simultaneously spontaneous discharge at too short distances was avoided. The above experiments show operation at high voltage and low current. Although useful for some applications, many applications will benefit from low-voltage and high-operating current. From the equality ½ mv 2 =qV target , it follows that this can be achieved by increasing droplet charge density q/m . Using inductive charging and a more conductive 0.1 M KCl solution, we could operate a single pore at 500 V target voltage and 50 nA current with 12% efficiency ( Fig. 2e,f ). The droplet charge density obtained in these microdroplets was about half the Rayleigh limit (the Rayleigh limit describes the droplet charge at which Coulomb repulsion overcomes surface tension and droplets become unstable. It equals Coulomb, where σ is the surface tension (0.07 N m −1 for water), ɛ 0 the permittivity of free space and d the droplet diameter.). An analysis of the experiments with 10 μm diameter pores indicated that the largest losses occur in the acceleration phase due to pore friction and jet surface formation energy ( Supplementary Note 1 ). Both can be substantially reduced by using a larger pore diameter. To still decelerate the heavier droplets at practical target potentials (<20 kV), a larger droplet charge needs to be induced. Experiments were performed with a 30-μm pore in combination with inductive charging by a guard ring voltage using a more conductive 10 mM KCl solution. Figure 3a,b shows the results of two experiments, plotting currents and efficiency against induction voltage. They show a maximum conversion efficiency of 48%. Figure 3: Two experiments using a 30-μm diameter pore. ( a ). Currents I 1 and I 2 as a function of gate voltage. ( b ) Efficiency as a function of gate voltage with a 1.01-TΩ load resistance. Applied pressure 1.38 bar, average flow rate 6.55 μl s −1 , solution 10 mM KCl, target distance 2.5 cm (experiment 1) and 2.0 cm (experiment 2). Full size image The conversion method demonstrated here is superficially similar to but fundamentally different from the Kelvin droplet generator, or ‘Kelvin’s thunderstorm [22] , [23] . In the Kelvin droplet generator, the action of gravity opposes the electrical force ( mg=−qE ), whereas in our ballistic system inertia opposes the electrical force ( ma=−qE ). This fundamentally different physics, coupled to the orders of magnitude higher charge densities q/m obtainable in microdroplets (~10 4 times higher than in Kelvin’s drops) offers the great practical advantage that we can work at 10 4 g instead of 1 g. By obtaining the energy from velocity rather than mass, 10 4 times lower volume flow rates can be used, strongly increasing the practical usefulness of the device. Inspired by the Kelvin generator, we also successfully operated a self-excited ballistic device with two membranes and targets, with each target connected to the guard ring under the opposite membrane, and obtained an efficiency of 18%. A paper on this work is in preparation. Ballistic energy conversion has myriad practical applications. A remarkable property of this conversion method is the very high-power density obtained, which is much higher than with any classical conversion method. The total power is conveniently scalable by increasing the pore number using MEMS (MicroElectroMechanical Systems) techniques [24] and if scaling holds up, 160 kW could be obtained on 1 m 2 footprint. Direct practical use could be in high-voltage microfluidics [25] . Ten thousand pores, for example, will increase the current to 50 μA and the load impedance to 10 MΩ, values suitable for microchip capillary electrophoresis. Additional engineering targets can be to reduce the hydrodynamic pore resistance and to increase droplet monodispersity. For the development of practically useful systems, a number of significant technical challenges will need to be overcome. Upscaling the design to large pore numbers is not a straightforward task, as medium to high voltages are used in combination with a high water throughput. The use of a porous membrane gives the risk of clogging, which necessitates high-quality filtering. Clogging may lead to dripping, which can give rise to wetting of the chip holder, short circuiting guard ring and water reservoir. Deposition of a hydrophobic anti-wetting coating is a possible engineering approach to this issue. Finally, continuous operation of a multipore design at high-flow volume rates in a small package will necessitate the incorporation of structures for liquid collection. Interestingly, the inverse procedure of the one used here, namely, the acceleration of charged droplets by an applied electrical field, is used for many and diverse applications such as electrostatic painting and printing [26] , colloid thrusters fluorescence-activated cell sorting [27] , electrospray ionization [28] and colloid thrusters [29] . We expect that these applications will benefit greatly from the newly gained physical insights. Pressure and electronic measurement set-up Figure 1a schematically shows the experimental set-up. A silicon nitride membrane with a single cylindrical pore of 10 or 30 μm diameter was mounted in a poly(methyl methacrylate) reservoir using rubber O-rings. A platinum electrode sputtered on the backside of the chip was connected to ground via a picoammeter (Keithley 6485) to measure the current from ground to electrode ( I 1 ). The reservoir was filled with purified water or KCl solution, which were expelled through the pore using a pressurized gas source (99% N 2 ) controlled with a pressure regulator (Norgren R07-100-RNKG) and with a pressure sensor (Sensortechnics CTE 8016 GY7). A particle filter (2 μm) was placed in the fluid line for particle filtration. The volume flow rate was measured by a flow meter (Bronkhorst Mini Cori M12). Guard ring and prevention of discharge A piece of aluminium foil (less than 0.1 mm thickness) with a 2-mm diameter hole was placed as metal guard ring at 1.5 mm (10 μm pore) or 5.0 mm (30 μm pore) from the exit. The ring could be maintained at ground potential or at a negative potential by inserting a voltage source between ground and ring. In some experiments, the current was measured from ground to the ring ( I 3 ) using a multimeter in the voltage range. The droplets generated by the break-up of the liquid jet were collected on a hollow stainless steel target, on the inside connected to a high-voltage cable (HSW Silicone cable) to prevent corona discharge. The cable was connected to ground via series-connected load resistors. The resistors were immersed in insulating oil (Shell Diala S2-ZU-I) to prevent losses by corona discharge ( Supplementary Fig. 9 ). At the grounded terminal, a series-connected picoammeter (Keithley 6487) measured the current ( I 2 ) from target to ground. The measurement data are tabulated in Supplementary Tables 1 and 3 . How to cite this article: Xie, Y. et al . High-efficiency ballistic electrostatic generator using microdroplets. Nat. Commun. 5:3575 doi: 10.1038/ncomms4575 (2014).